A top–down strategy towards monodisperse colloidal lead sulphide quantum dots Monodisperse colloidal quantum dots with size dispersions <10% are of great importance in realizing functionality manipulation, as well as building advanced devices, and have been normally synthesized via ‘bottom–up’ colloidal chemistry. Here we report a facile and environmentally friendly ‘top–down’ strategy towards highly crystalline monodisperse colloidal PbS quantum dots with controllable sizes and narrow dispersions 5.5%< σ <9.1%, based on laser irradiation of a suspension of polydisperse PbS nanocrystals with larger sizes. The colloidal quantum dots demonstrate size-tunable near-infrared photoluminescence, and self-assemble into well-ordered two-dimensional or three-dimensional superlattices due to the small degree of polydispersity and surface capping of 1-dodecanethiol, not only serving as a surfactant but also a sulphur source. The acquisition of monodisperse colloidal PbS quantum dots is ascribed to both the quantum-confinement effect of quantum dots and the size-selective-vaporization effect of the millisecond pulse laser with monochromaticity and low intensity. Owing to quantum-confinement effects (QCE), semiconductor nanocrystals (quantum dots, QDs) exhibit attractive size-tunable electrical and optical properties, which make them highly desirable in the applications of optoelectronics and biotechnology [1] , [2] , [3] , [4] , [5] , [6] , [7] . Because of the striking size-dependence of characteristics, monodisperse QDs, with a size dispersion (or polydispersity) σ <10% ( [8] ), are of great importance in realizing functional control and manipulation, such as achieving very sharp photoluminescence and a precise tuning of the emission by varying QDs sizes [9] . Moreover, monodisperse colloidal QDs have been regarded as promising building blocks for advanced crystal superlattices and devices with abnormal electrical and optical behaviours, resulting from the quantum mechanical and dipolar interactions between nanocrystal units [10] . General synthesis approaches towards monodisperse colloidal QDs have primarily employed solution-phase colloidal chemistry (the so called ‘bottom–up’ strategy), where an effective separation of nucleation and growth steps is believed to be the key in obtaining monodisperse nanoparticles [11] . Specifically, several ‘bottom–up’ approaches have been developed for preparing monodisperse colloidal PbS QDs, including the most popular organic-phase hot-injection technique [12] , [13] , [14] , which induces burst nucleation by a rapid injection of excess precursor(s) into a hot surfactant solution. A ‘top–down’ approach, laser fragmentation in liquid, has been normally adopted to realize size-reduction and size-distribution-narrowing of colloidal noble metal (gold and silver) nanoparticles, through nanosecond laser vaporization [15] , [16] , [17] or picosecond-laser-induced Coulomb explosion [18] of nanoparticles upon laser irradiation. However, the polydispersity after laser treatments usually remains fairly large ( σ >10%). It was not until very recently that Werner et al . [19] achieved a polydispersity of 6.1% by applying high pressures during nanosecond laser irradiation of colloidal gold nanoparticles. Hitherto, the ‘top–down’ strategy has never been used in acquiring monodisperse colloidal semiconductor nanocrystals, although some attempts have been made lately in the cases of Se [20] , ZnO [21] , and Si [22] QDs with polydispersity σ >15%. Different from fast and ultrafast lasers, long-pulse lasers, that is, millisecond-pulse lasers, posses rather low power densities, which usually cause linear absorption [23] and Joule heating [24] of the target. On the other hand, the band gap of QDs widens as QDs size reduces due to QCE. Therefore, when a long-pulse monochromatical laser is employed to irradiate polydisperse colloidal QDs, those with large sizes and band gaps narrower than the photon energy can be heated and even evaporated, while those with small sizes and wider band gaps are transparent and keep intact, giving rise to monodisperse QDs in a top–down way. As an example, in the present work, monodisperse colloidal PbS QDs are prepared with controllable sizes (3.5~5.5 nm) and narrow dispersions (5.5%< σ <9.1%), simply by means of millisecond laser irradiation of a suspension of polydisperse raw PbS nanocrystals with relatively large sizes (that is, tens of nanometres). The size control of QDs is realized by an adjustment of the water-bath temperature from 0–30 °C and the as-prepared PbS QDs exhibit size-tunable near-infrared (NIR) photoluminescence. Quantitative experimental studies on QDs size evolution with laser ablation duration and a theoretical calculation of complete vaporization threshold confirm that the acquisition of monodisperse QDs arise from both the robust QCE-induced band gap wideness and the selective vaporization of nanocrystals by low-intensity laser beam. To the best of our knowledge, this is the first report on the top–down synthesis of monodisperse colloidal QDs with σ <10%. This facial top–down synthetic route manifests itself as an environmentally friendly method in terms of not only employing low-temperature conditions (0~30 °C), but also involving a low-toxic lead target and 1-dodecanethiol (DDT, C 12 H 26 S). Our strategy is potentially universal for the synthesis of monodisperse colloidal QDs with prominent QCE, such as CdSe, PbSe, PbTe and so on. Synthesis of monodisperse PbS QDs Monodisperse colloidal PbS QDs were prepared by adopting a two-step laser ablation/irradiation route ( Supplementary Fig. S1a,b ). In this process, raw PbS nanocrystals were first produced by laser ablation of a lead plate in DDT, which showed a polydisperse size distribution varying from 20–50 nm ( Supplementary Fig. S2a ), and the rock salt structure of PbS nanocrystals (ICCD-5-592) were confirmed by the X-ray diffraction pattern ( Supplementary Fig. S2b ). Afterwards, the second laser treatment (irradiation duration t =20 min, water-bath temperature T b =30 °C) produced PbS QDs with a significant size-reduction and uniformity in both the top ( Fig. 1a ) and bottom ( Supplementary Fig. S3 ) of solution. A statistical analysis on more than 300 nanoparticles in transmission electron microscope (TEM) images demonstrates that the as-prepared nanoparticles are highly monodisperse with diameters of 5.5±0.3 nm ( σ =5.5%) (inset of Fig. 1a ). Besides, the nanoparticles self-assembled into a two-dimensional hexagonal superlattice on the copper grid, also indicative of a high degree monodispersity of the nanoparticles. The diffraction rings shown in the selected area electron diffraction pattern of the nanoparticles ( Fig. 1b ) index well to the cubic rock salt structure of bulk PbS. The high-resolution TEM image of one of the nanoparticles ( Fig. 1c ) reveals its high-crystalline nature with a lattice spacing of 0.295 nm, expected for d 200 of bulk PbS crystals (ICDD-5-592), and the corresponding fast-Fourier transform pattern (inset of Fig. 1c ) implies the face-centered cubic phase oriented along [001] direction. Moreover, energy-dispersive X-ray spectroscopy spectrum ( Supplementary Fig. S3 ) proves that the nanoparticles contain Pb and S atoms, whereas the signals of C and Cu ought to arise from the carbon coated copper grid. In the case of colloids with relatively high concentrations, the PbS QDs could form a three-dimensional hexagonal-close-packed superlattice assembly ( Supplementary Fig. S4 ). 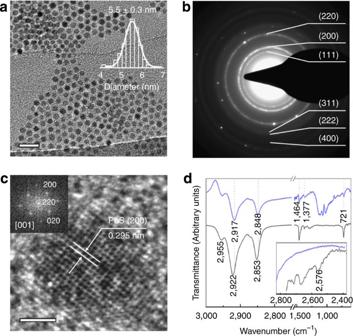Figure 1: PbS QDs produced at water-bath temperature 30 °C. (a) TEM image by laser irradiation of raw PbS nanocrystals for 20 min. Scale bar, 20 nm. Inset displays size histogram of QDs and corresponding Gaussian fit. (b) Selected area electron diffraction pattern of PbS QDs shown ina, where labelled diffraction rings match well with PbS face-centered cubic phase. (c) High-resolution TEM image of one of the QDs shown ina. The scale bar represents 2 nm, and the inset is the corresponding fast-Fourier transform pattern. (d) Fourier transform-infrared spectra of PbS quantum dots coated with DDT (top) and neat/pure DDT (bottom). Note that the top curve is magnified 12 times for clarification of the absorption peaks. The inset shows enlarged spectra in the regime of 2,825~2,930 cm−1. The main absorption peaks arise from the asymmetric vibration of CH3(2,955 cm−1), the asymmetric (2,922 cm−1) and symmetric stretching of CH2(2,853 cm−1), the CH2scissoring mode (1,464 cm−1), the CH3symmetric bending vibration (1,377 cm−1) and the CH2rocking band (721 cm−1) (25). Figure 1: PbS QDs produced at water-bath temperature 30 °C. ( a ) TEM image by laser irradiation of raw PbS nanocrystals for 20 min. Scale bar, 20 nm. Inset displays size histogram of QDs and corresponding Gaussian fit. ( b ) Selected area electron diffraction pattern of PbS QDs shown in a , where labelled diffraction rings match well with PbS face-centered cubic phase. ( c ) High-resolution TEM image of one of the QDs shown in a . The scale bar represents 2 nm, and the inset is the corresponding fast-Fourier transform pattern. ( d ) Fourier transform-infrared spectra of PbS quantum dots coated with DDT (top) and neat/pure DDT (bottom). Note that the top curve is magnified 12 times for clarification of the absorption peaks. The inset shows enlarged spectra in the regime of 2,825~2,930 cm −1 . The main absorption peaks arise from the asymmetric vibration of CH 3 (2,955 cm −1 ), the asymmetric (2,922 cm −1 ) and symmetric stretching of CH 2 (2,853 cm −1 ), the CH 2 scissoring mode (1,464 cm −1 ), the CH 3 symmetric bending vibration (1,377 cm −1 ) and the CH 2 rocking band (721 cm −1 ) ( [25] ). Full size image Fourier transform-infrared (FTIR) measurements reveal that, in contrast to free DDT, the S-H stretching vibration band at 2576, cm −1 is absent in the spectrum of capped QDs (inset of Fig. 1d ), suggesting that the S-H bond is broken and the DDT molecules are chemisorbed as thiolates onto the surface of PbS QDs in a monodentate manner [25] . Meanwhile, the asymmetric and symmetric CH 2 stretching bands of the coated nanocrystals locate at lower wavenumbers (2917 and 2848, cm −1 , respectively), compared with free DDT ( Fig. 1d ). As illustrated in a number of publications [26] , [27] , the position of the methylene stretching vibrations has been commonly adopted as an indicator of the order (crystallinity) of the alkyl chains, and such a redshift from the free thiols infers that the chemisorbed DDT molecules are of a higher degree of ordering on the surface of the QDs. Hence, DDT serves as not only a sulphur source, but also a coordinating solvent that prevents QDs growth and agglomeration. Effect of the reaction temperature The size of monodisperse PbS QDs can be precisely tuned by adjusting the temperature of water-bath, T b . Besides T b =30 °C, the second laser irradiation was also carried out at T b =0, 20, 50 and 70 °C, for 20 min. The as-obtained products at lower temperatures appear to be quasi-spherical with uniform sizes ( Fig. 2a ), that is, 4.4±0.4 nm ( σ =9.1%) and 3.5±0.3 nm ( σ =8.6%) for T b =20 and 0 °C, respectively ( Fig. 2b ). Figs 1a and 2a demonstrate clearly a drastic reducing of the mean diameter of QDs with decreasing T b . However, as T b further increases to 50 and 70 °C, a ripening of QDs becomes dominant in the final products, giving rise to polydisperse non-spherical nanocrystals ( Supplementary Fig. S5a,5b ). However, we might be able to further increase the range of monodisperse nanocrystals sizes by adopting appropriate stabilizing agents for higher temperatures, which is still in progress. 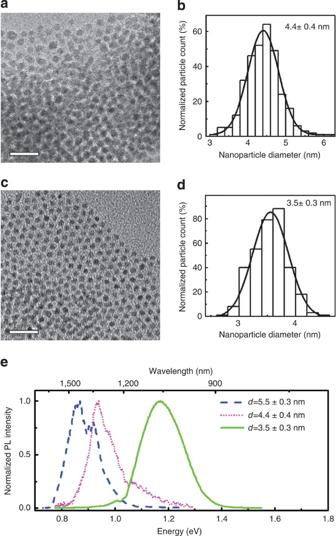Figure 2: PbS QDs produced at different water-bath temperatures. TEM images of samples produced by laser irradiation for 20 min ata, 20 °C andc, 0 °C. Scale bars, 20 nm. Size histograms of QDs prepared atb, 20 °C andd, 0 °C, and corresponding Gaussian fits. (e) Normalized room-temperature photoluminescence spectra of PbS QDs with respective diametersd, with an excitation wavelength of 400 nm. The discernable feature around 1,400 nm (0.9 eV) of the dashed curve could be attributed to the absorption by atmospheric water vapor14. The as-produced PbS QDs display strong and size-tunable photoluminescence in the NIR spectral regime, as seen in Fig 2e . Because to QCE, the emission peaks exhibit an obvious blue-shift as QDs get smaller, namely, the 5.5 nm, 4.4 nm and 3.5 nm PbS QDs show luminescence at 1,427 nm (0.87 eV), 1,320 nm (0.94 eV) and 1,060 nm (1.17 eV), respectively, and the full widths at half-maximum height of the photoluminescence spectra of respective QDs are 130 meV, 104 meV and 187 meV, in good accord with recently reported literature data [14] . Figure 2: PbS QDs produced at different water-bath temperatures. TEM images of samples produced by laser irradiation for 20 min at a , 20 °C and c , 0 °C. Scale bars, 20 nm. Size histograms of QDs prepared at b , 20 °C and d , 0 °C, and corresponding Gaussian fits. ( e ) Normalized room-temperature photoluminescence spectra of PbS QDs with respective diameters d , with an excitation wavelength of 400 nm. The discernable feature around 1,400 nm (0.9 eV) of the dashed curve could be attributed to the absorption by atmospheric water vapor [14] . Full size image Effect of the laser ablation duration We performed quantitative investigations on the effect of laser ablation duration ( t ) on the evolution of average size of PbS QDs prepared at T b =0 °C. As seen in Fig. 3 , at t =1 min, raw PbS nanocrystals with sizes of tens of nanometres are dramatically converted to fairly small PbS QDs with a mean diameter of 4.9±0.8 nm. Meanwhile, as laser irradiation time extends, the average size of as-prepared PbS QDs reduces monotonically until reaching a minimum limit of 3.5±0.3 nm at around t =20 min. At the same time, the degree of polydispersity in the QDs also decreases, changing from~16.0–8.6%, with prolonged irradiation (inset of Fig. 3 ). Consequently, laser irradiation of raw PbS nanocrystals can effectively reduce the average size and size dispersion, and finally results in monodisperse QDs. Similar trends also applies to the cases of elevated water-bath temperatures, for example, T b =30 °C, where 8 min of laser irradiation of QDs achieves a minimum size limit of 5.5 nm, and an extension of t to 20 min lowers the size dispersion from 9.1% (5.5±0.5 nm) to 5.5% (5.5±0.3 nm), while keeping the average QDs size unchanged. 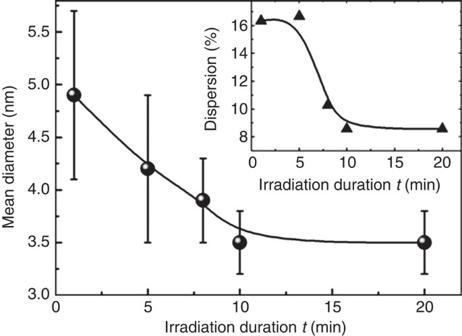Figure 3: Evolution of the mean diameter of PbS QDs with laser ablation duration. The water-bath temperature is 0 °C, and the inset shows the evolution of respective size dispersion of QDs with ablation duration. Figure 3: Evolution of the mean diameter of PbS QDs with laser ablation duration. The water-bath temperature is 0 °C, and the inset shows the evolution of respective size dispersion of QDs with ablation duration. Full size image The generation of raw PbS nanocrystals by laser ablation of a lead target immerged in DDT follows the typical growth mechanism of nanoparticles in millisecond laser ablation [28] . On the other hand, the size-reduction of the raw nanocrystals upon laser irradiation may result from two possible mechanisms, namely, the heating-melting-vaporization of nanoparticles and Coulomb explosion (photofragmentation induced by electron ejections). As the millisecond pulse laser we used is a relatively slow laser with low intensity (10 7 W cm −2 , at most), the latter mechanism should be ineffective here and the heating-melting-vaporization model dominates [24] , [29] . Meanwhile, linear absorption is the main absorption process of long-pulse laser energy by targets [23] , therefore, PbS nanocrystals with band gap energies lower than 1.17 eV, the laser’s photon energy, can be heated by laser pulses through Joule heating, while those with larger band gaps can hardly. Consequently, the strong QCE in PbS QDs can induce a ‘selective heating of nanocrystals’ phenomenon during laser irradiation, and the minimum size of PbS QDs that could be heated is thus estimated to be d* =3.6 nm, according to the reported relation between the PbS QDs band gap and the particle size [30] . To actualize a full vaporization of a PbS nanoparticle with a certain diameter ( d 0 ), the laser fluence must exceed a threshold, J* , which were calculated by adopting Equation (1) ( [29] ), where the physical constants of PbS, i.e. , the density ρ , heat capacity c p , boiling temperature T bl , melting heat ΔH m , and boiling heat ΔH b were adopted from Lange [31] . ΔQ c , and ΔQ r represent heat loss due to convection and radiation [32] , respectively, which could not be neglected due to relatively long-pulse duration herein, τ =5 ms. , per particle absorption cross-section at 1,064 nm (laser wavelength) could be modelled by the Maxwell-Garnett effective medium theory [33] ( Fig. 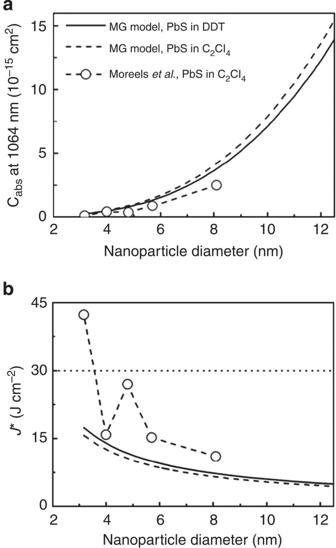Figure 4: Laser fluence threshold for the full vaporization of a PbS nanoparticle. (a) Absorption cross-section at 1064, nm as a function of size for PbS nanoparticles dispersed in DDT (—,n=1.46) and C2Cl4(---,n=1.53), calculated by Maxwell-Garnett effective medium theory, as well as experimental data (-O-) for PbS QDs in C2Cl4by Moreelset al.33,35. (b) Corresponding complete vaporization threshold calculated using Equation (1) given in the text. 4a ), with the dielectric function of bulk PbS at 1,064 nm ( ε =18.8+4.57i) ( [34] ) and the DDT refractive index ( n =1.46), Figure 4: Laser fluence threshold for the full vaporization of a PbS nanoparticle. ( a ) Absorption cross-section at 1064, nm as a function of size for PbS nanoparticles dispersed in DDT (—, n =1.46) and C 2 Cl 4 (---, n =1.53), calculated by Maxwell-Garnett effective medium theory, as well as experimental data (-O-) for PbS QDs in C 2 Cl 4 by Moreels et al . [33] , [35] . ( b ) Corresponding complete vaporization threshold calculated using Equation (1) given in the text. Full size image where d 0 in nanometres. However, it should be noted that the size quantization effects become substantial at energies (that is, 1.17 eV) not far above the band edge of PbS QDs [35] . Consequently, might be slightly overestimated in the Maxwell-Garnett model, particularly for small QDs, as demonstrated in the case of C 2 Cl 4 as solvent ( n =1.53), compared with the experimental data [33] , [35] ( Fig. 4a ). Owing to lack of experimental examinations of in the case of DDT as solvent, we adopted Moreels’ data [33] , [35] , for the refractive index of C 2 Cl 4 close to that of DDT, to calculate the complete vaporization threshold J* by using Equation (1), where for convective and radiative heat loss estimations, the convection heat transfer coefficient h and emissivity ε were set as 5 and 0.05, respectively. As displayed in Fig. 4b , the laser fluence used in our case (30 J cm −2 ) is high enough to guarantee a complete vaporization of PbS nanocrystals with band gap energies lower than that of the laser photons (1.17 eV). On account of the above, the formation mechanism of monodisperse PbS QDs is proposed and summarized in Fig. 5 . When the polydisperse PbS nanocrystals are exposed to the millisecond laser pulse with wavelength of 1064, nm (1.17 eV), nanoparticles with large sizes ( d 0 ≥ d* ) and narrow band gaps ( E g ≤1.17 eV) absorb the incident light and are heated effectively, while those with smaller sizes ( d 0 < d* ) are transparent to the infrared laser due to QCE-induced band gap wideness ( Fig. 5a ). Because of the high enough laser fluence, all of the heated nanoparticles are vaporized completely, while the smaller ones keep intact, leading to a selective vaporization of nanocrystals ( Fig. 5b ). The subsequent condensation of the nanometer-sized hot clouds of vaporized Pb/S atoms causes the formation of smaller PbS nanoparticles, which includes nucleation and following growth process. The rapid vaporization of PbS nanoparticles in liquid medium by laser pulses produces a high degree of supersaturation of monomers and results in ‘burst nucleation’. The nuclei grow by collecting remaining monomers, which diffuse to them through the solution, and finally reach an equilibrium size due to a complete coating of a DDT layer. As irradiation duration extends, more and more PbS nanoparticles are heated, vaporized and transformed into smaller ones ( Fig. 5c ). Thus PbS nanoparticles become smaller and more uniform with prolonged irradiation, as shown in Fig. 3 , and finally monodisperse PbS QDs with average size of 3.5 nm ( σ =8.6%), slightly smaller than d* , are achieved in the case of T b =0 °C ( Fig. 5d ). For elevated water-bath temperatures, that is, T b =20 and 30 °C, we preliminarily infer that the diffusion of PbS monomers accelerate at higher temperatures, while the adsorption of DDT on the surface of nanoparticles weakens. As a result, newly formed nanoparticles grow much faster and the equilibrium QDs size would be increased with ambient temperatures and larger than d* (see Figs 1a and 2a ). 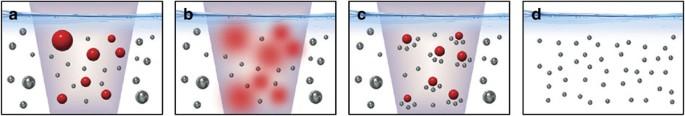Figure 5: Schematic illustration of the formation of monodisperse PbS QDs. (a) Selective heating of large nanoparticles. (b) Vaporization of heated nanoparticles. (c) Condensation of hot clouds of vaporized Pb/S atoms and further selective heating of smaller nanoparticles with the size over the threshold (d*). (d) Formation of monodisperse PbS QDs. Figure 5: Schematic illustration of the formation of monodisperse PbS QDs. ( a ) Selective heating of large nanoparticles. ( b ) Vaporization of heated nanoparticles. ( c ) Condensation of hot clouds of vaporized Pb/S atoms and further selective heating of smaller nanoparticles with the size over the threshold ( d* ). ( d ) Formation of monodisperse PbS QDs. Full size image In order to confirm the size selectivity due to QCE-induced band gap wideness, nearly monodisperse CdSe QDs, another class of important visible optoelectronic semiconductors with band gap energy larger than that of PbS, were fabricated preliminarily via the laser irradiation technique using 532 nm nanosecond laser (6 ns, 0.5 J cm −2 ). Based on the correlation of CdSe band gap energy and its particle size [36] , the minimum size of CdSe QDs that could be heated by laser with photon energy of 2.33 eV is d* CdSe =2.7 nm. On the other hand, the complete vaporization threshold J* CdSe of laser was calculated to be 0.4 J cm −2 , lower than that of the laser we used, by adopting Equations (1), (2), and the experimental data of absorption cross-section of CdSe QDs [37] . Therefore, analogous to the case of PbS, CdSe QDs with diameters of 2.6±0.4 nm ( Supplementary Fig. S6a ) were acquired after laser irradiation of a suspension of raw CdSe nanocrystals with polydisperse sizes from tens to hundreds of nanometres ( Supplementary Fig. S6b ) dispersed in oleic acid solution at T b =0 °C. The size dispersion σ of CdSe QDs could be further improved by more detailed studies on the selection of surfactant solutions. The QDs are highly crystallized as exhibited in the high-resolution TEM image (top inset of supporting Supplementary Fig. S6a ), where the lattice spacing of 0.198 nm corresponds to the (103) plane of hexagonal CdSe (ICCD-77-2307). Meanwhile, the selected area electron diffraction pattern of the nanoparticles (bottom inset of supporting Supplementary Fig. S6a ) indexes well to the hexagonal structure of bulk CdSe. In conclusion, we have demonstrated a facile and environmentally friendly ‘top–down’ strategy towards highly crystalline monodisperse colloidal PbS QDs (5.5%< σ <9.1%) by means of laser irradiation. The size control of QDs ranging from 3.5–5.5 nm was achieved by tuning the water-bath temperature from 0–30 °C, and the as-produced QDs displayed strong and size-tunable NIR luminescence. Quantitative experimental studies on the size evolution of QDs with laser ablation duration and preliminary theoretical analyses on the complete vaporization threshold implied that our strategy towards monodisperse colloidal QDs was primarily based on both the robust QCE-induced band gap wideness and the selective vaporization of nanocrystals by low-intensity laser beam, thus potentially a universal synthetic strategy for monodisperse colloidal QDs with prominent QCE, such as CdSe, PbSe, PbTe and so on. Preparation of PbS QDs We synthesized monodisperse colloidal PbS QDs by adopting a two-step laser ablation/irradiation route ( Supplementary Fig. S1a,b ). First, raw PbS nanocrystals were prepared by laser ablation of a lead target in reactive liquid medium. Particularly, a pure lead plate supported by a target holder was immersed in DDT with a thin liquid layer (thickness 5 mm) above the target surface, and ablated by the first harmonic (wavelength 1,064 nm) of millisecond pulsed Nd:YAG laser (pulse width 2 ms, repetition rate 2 Hz, pulse energy~4 J per pulse, focal spot diameter 0.2 mm), focused onto the target surface, for a while until the colour of solution turned black. During ablation, the solution was kept stirring with a magnetic stirrer and the irradiated spot was moved around occasionally. The whole set-up could guarantee a considerably high yield of nanoparticles. Raw PbS nanocrystals were separated from the as-obtained black colloid by centrifugation, rinsed with ethanol, dried, weighed and redispersed in DDT to make a 4.3 mM of suspension. In the second step, 0.25 ml of the as-prepared raw PbS nanocrystals dispersion (0.43 mM) was transferred to a quartz cell with an inner diameter of 10.0 mm and irradiated by the unfocused laser (pulse width 5 ms, repetition rate 2 Hz, spot diameter 8.0 mm, pulse energy density ~30 J cm −2 ) for a period of time t (1~20 min). The temperature of the colloid solution was controlled via a water-bath ( T b =0~30 °C). A relatively uniform irradiation of the colloidal nanocrystals could be guaranteed, for the inner diameter of the cell slightly larger than the laser-spot size. During the irradiation, a significant colour change of the colloid from opaque black to transparent light grey was observed, indicative of the formation of small PbS QDs. Characterization TEM images were acquired by using an FEI Technai G2 F20 transition electron microscope equipped with a field-emission gun. The compositions of the products were determined by an Oxford INCA energy-dispersive X-ray spectroscopy module attached to the TEM. A Hitachi S-4800 scanning electron microscope was used to perform morphology observations of the raw nanocrystals. Powder X-ray diffraction measurements were carried out on a Rigaku D/max 2500v/pc diffractometer. The UV–vis-NIR absorption spectra were obtained with a Hitachi U-4100 spectrophotometer. Near-infrared photoluminescence measurements were performed on a fluorescence spectrometer (FL3-221-TCSPC, HORIBA Jobin Yvon Inc) with a 450-W xenon lamp and a photomultiplier tube as detector working in a photon counting mode. Infrared spectra of samples were recorded using a Bruker Tensor 27 FT-IR spectrometer in the range of 400~4,000 cm −1 . How to cite this article: Yang, J. et al . A top–down strategy towards monodisperse colloidal lead sulphide quantum dots. Nat. Commun. 4:1695 doi: 10.1038/ncomms2637 (2013).